TheGonium pectoralegenome demonstrates co-option of cell cycle regulation during the evolution of multicellularity The transition to multicellularity has occurred numerous times in all domains of life, yet its initial steps are poorly understood. The volvocine green algae are a tractable system for understanding the genetic basis of multicellularity including the initial formation of cooperative cell groups. Here we report the genome sequence of the undifferentiated colonial alga, Gonium pectorale, where group formation evolved by co-option of the retinoblastoma cell cycle regulatory pathway. Significantly, expression of the Gonium retinoblastoma cell cycle regulator in unicellular Chlamydomonas causes it to become colonial. The presence of these changes in undifferentiated Gonium indicates extensive group-level adaptation during the initial step in the evolution of multicellularity. These results emphasize an early and formative step in the evolution of multicellularity, the evolution of cell cycle regulation, one that may shed light on the evolutionary history of other multicellular innovations and evolutionary transitions. Multicellular organisms have independently evolved numerous times throughout the tree of life including plants, animals, fungi, cyanobacteria, amoeba, brown algae, red algae and green algae [1] , [2] . In animals, multicellularity emerged 600–950 million years ago (Myr ago) correlating with a large expansion of genes encoding transcription factors, signalling pathways, and cell adhesion genes that were co-opted from their unicellular ancestors [3] , [4] Similarly, multicellular, terrestrial plants emerged ∼ 750 Myr ago correlating with an expansion of many signalling pathways present in their unicellular relatives [5] , [6] . However, because most multicellular lineages have long diverged from their unicellular relatives, the genomic signature of the transition to multicellularity has been obscured, and consequently this evolutionary process remains enigmatic. The volvocine green algae are a unique model system for the evolution of multicellularity because the unicellular ancestry is clear, the emergence of multicellularity occurred ∼ 230 Myr ago, and species exhibit a stepwise increase in morphological complexity ranging from undifferentiated colonies to differentiated multicellular species [7] , [8] ( Fig. 1 , Supplementary Figs 1,2 ). Unicellular Chlamydomonas reinhardtii is thought to resemble the unicellular ancestor of multicellular volvocines, including undifferentiated Gonium pectorale and differentiated Volvox carteri ( Fig. 1 ). 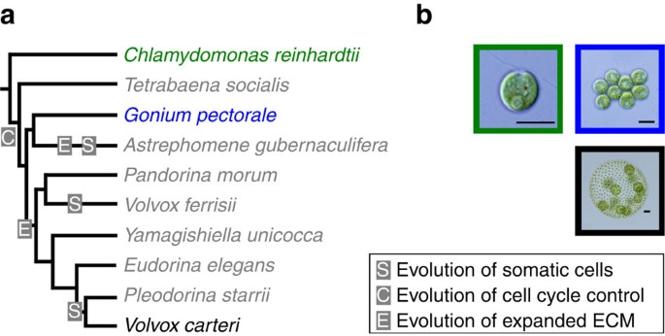Figure 1: Volvocine phylogenetic tree. (a) Evolution of cell cycle control (C), expanded ECM (E) and somatic cells (S) are denoted. (b) Micrographs ofChlamydomonas(green; scale bar, 10 μm),Gonium(blue; scale bar, 10 μm) andVolvox(black; scale bar, 25 μm) show morphological differences. Figure 1: Volvocine phylogenetic tree. ( a ) Evolution of cell cycle control (C), expanded ECM (E) and somatic cells (S) are denoted. ( b ) Micrographs of Chlamydomonas (green; scale bar, 10 μm), Gonium (blue; scale bar, 10 μm) and Volvox (black; scale bar, 25 μm) show morphological differences. Full size image Chlamydomonas undergoes a variant cell cycle ( Supplementary Fig. 2 ), regulated by homologues of the retinoblastoma cell cycle pathway, termed multiple-fission where it divides by a series of rapid cell divisions producing individual daughter cells [9] , [10] , [11] . Gonium typically forms 8- or 16-celled undifferentiated colonies, where each constituent cell resembles a Chlamydomonas cell ( Fig. 1 ). Gonium also undergoes multiple fission forming daughter colonies by keeping cells attached after multiple-fission, suggesting either cell cycle regulation [12] , or cell–cell adhesion has been modified to promote multicellularity. In Gonium , like Chlamydomonas , growth and cell division are uncoupled [13] , [14] . Asexual juvenile Gonium colonies grow (without cell division) into adults. After cell division through multiple-fission, juvenile colonies hatch forming 8 or 16 daughter colonies of 8 or 16 cells ( Supplementary Fig. 2 ). Volvox contains approximately 2,000 small, terminally differentiated, somatic cells on the surface of the spheroid and approximately 16 large reproductive cells embedded in extracellular matrix (ECM) inside the spheroid ( Fig. 1 ). Volvox also has modified multiple fission where germ–soma separation is established after an asymmetric cell division [8] , [14] . The transition to multicellularity in the Volvocales was thought to involve at least 12 steps ( Supplementary Fig. 1 ) [15] , [16] though the genetic basis of these steps remains enigmatic. Genomic comparison of the extremes of morphological complexity, Chlamydomonas and Volvox , suggests few genetic changes are required [17] , but it is unclear how and when the genes important for multicellularity evolved during these 12 steps [14] . By sequencing the genome of the undifferentiated, chlorophycean Gonium pectorale , a species without a differentiated ancestor [16] , we find co-option of cell cycle regulation, which occurred during the initial transition to cell groups, as the genetic basis for the evolution of multicellularity. The cell cycle regulation found in undifferentiated Gonium , co-opted in a multicellular context and shared with germ–soma-differentiated Volvox , indicates group-level adaptations in undifferentiated colonies. The early co-option of cell cycle regulation for group-level life cycle and reproduction is a critical and formative step in the evolution of multicellularity. Genomic comparisons of volvocine algae At the genomic level, the genomes of Chlamydomonas , Gonium and Volvox are similar, though various measures of genome compactness correlate with cell number, consistent with a long-term increase in organismal size [18] , [19] . Chlamydomonas and Gonium have similar GC content near 64%, while Volvox has 56% GC ( Table 1 ). Otherwise, Chlamydomonas , Gonium and Volvox have decreasing gene densities of 159.6, 120.9 and 113.7 genes per megabase, with an increasing average intron length of 279, 349 and 500 base pairs, respectively. Although intron length increases with organismal complexity, the number of introns per gene ( Chlamydomonas, 7.46; Gonium , 6.5; Volvox 6.8, Table 1 ) does not. GC content, intron length and gene density correlate with morphological complexity. Table 1 Summary statistics for genome level analyses for Chlamydomonas , Gonium and Volvox . Full size table We next examined genome-wide evolution in all three species to better understand the genetic basis for the evolution of multicellularity. A prediction of lineage-specific genes [20] shows few genes correlate with the evolution of multicellularity in the Volvocales (phylostratum 7; PS7) with a maximum of 180–357 genes ( Fig. 2a ). This suggests that the evolution of multicellularity does not rely upon the evolution of de novo genes. Though gene regulation may be important during multicellular innovation, the diversity and abundance of transcription factors is similar in Chlamydomonas , Gonium and Volvox ( Fig. 2b , Supplementary Table 1 , Supplementary Fig. 3 ). Although enrichment of transcription factors can correlate with the evolution of multicellularity [3] , this is not always the case [21] ; we found that Gonium and Volvox have fewer transcription factors than in Chlamydomonas ( Fig. 2b ). These include PHD domains (transcription and chromatin binding), DNA binding transcription factors and histones ( Fig. 2b , Supplementary Tables 2 and 3 , Supplementary Fig. 3 ). 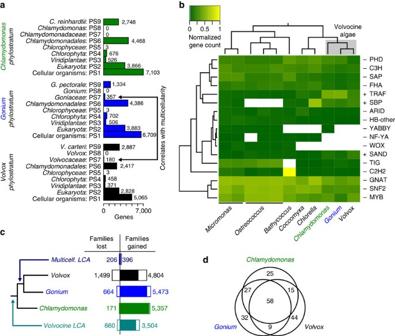Figure 2: Genome similarity in the Volvocales. (a) Predicted number of genes in each phylostratum (PS1–PS9) forChlamydomonas,GoniumandVolvox. (b) Heatmap of transcription factor abundance for all green algae. Significant over- (+) and under-representation (−) in colonial/multicellular lineages (GoniumandVolvox) is denoted (G test of independence,α=0.05). Rows are clustered (left), an accepted phylogeny is depicted (top). (c) Phylogenetic analysis of gene family evolution. Bars to the left and right of the vertical axis denote the lost and gained gene families respectively, relative to its parental node. (d) Venn diagram of the species distribution of Pfam A domains unique to the volvocine algae. Figure 2: Genome similarity in the Volvocales. ( a ) Predicted number of genes in each phylostratum (PS1–PS9) for Chlamydomonas , Gonium and Volvox . ( b ) Heatmap of transcription factor abundance for all green algae. Significant over- (+) and under-representation (−) in colonial/multicellular lineages ( Gonium and Volvox ) is denoted (G test of independence, α =0.05). Rows are clustered (left), an accepted phylogeny is depicted (top). ( c ) Phylogenetic analysis of gene family evolution. Bars to the left and right of the vertical axis denote the lost and gained gene families respectively, relative to its parental node. ( d ) Venn diagram of the species distribution of Pfam A domains unique to the volvocine algae. Full size image Using all published chlorophyte green algae genomes, we constructed Markov-based gene families ( Chlamydomonas , 73%; Gonium , 73%; Volvox , 70% of genes in gene families of size greater than one). Compared with 2,844 net gene families gained, which correlate with the origin of the Chlorophyceae, a phylogenetic analysis of these gene families suggests little protein innovation (110 net gene families) during the evolution of multicellularity ( Fig. 2c ). These same green algae genomes allowed analysis into Pfam domain innovation, which may correlate with the evolution of multicellularity. We found innovation of only nine Pfam domains correlating with the evolution of multicellularity ( Fig. 2d , Supplementary Table 4 ). 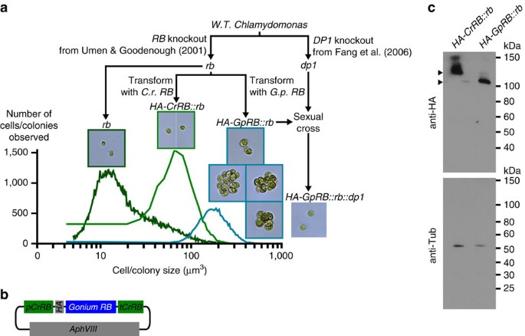Figure 4:Gonium RBcauses a colonial phenotype when expressed inChlamydomonas. (a) Transformation schematic showing resulting morphology overlaid onto cell and colony size measurements (logarithmic scale) of controlChlamydomonas RBmutant (rbormat3–4, transformed with empty vector), complementingHA-CrRB::rb(two of five independent transformations are shown) and colonialHA-GpRB::rb(four independent transformations are shown). Crossing colonialHA-GpRB::rbto aChlamydomonas DP1mutant (dp1) restores unicellularity inChlamydomonas(one of two independent matings are shown). (b) SchematicGonium RBtagged with 3XHA with its expression driven by theChlamydomonas RBpromoter and terminator11. (c) Anti-HA immunoblotting ofHA-CrRB::rbandHA-GpRB::rbwith anti-tubulin loading controls. Arrows indicate proteins at their expected molecular mass. Moreover, multicellular algae ( Gonium and Volvox ) have reduced Pfam domain diversity and abundance (compared with nine unicellular green algae, Supplementary Data 1 ); 394 Pfam A domains are significantly under-represented versus 129 over-represented Pfam domains ( Supplementary Fig. 4 ). Interestingly, there is an excess of species-specific genes ( Fig. 2a,c ) and Pfam domains ( Fig. 2d ) compared with multicellularity-correlated genes and Pfam domains, suggesting that species-specific adaptations are more numerous than changes correlating with the evolution of multicellularity. We observe more evidence of species-specific, rather than multicellular-specific, protein innovations, suggesting species-specific adaptation ( Fig. 2a,c,d , Supplementary Tables 5–8 ) rather than genome-wide differences correlating with the evolution of multicellularity. The evolution of multicellularity in the volvocine algae does not require large-scale genomic innovation. Co-option of cell cycle regulation for multicellularity Notably, we observe that the genetic innovation correlating with multicellularity, shared between Gonium and Volvox , evolved through co-option of existing developmental programs of cell cycle control. Volvocine algae have a common multiple-fission life cycle, with variation in timing and number of divisions ( Supplementary Fig. 1 ) [14] . Like most eukaryotes, including plants and animals, their cell cycles are regulated by homologues of the retinoblastoma cell cycle regulatory pathway ( Fig. 3 , Supplementary Figs 5–8 , Supplementary Table 9 ) [9] , [10] , in which cyclin-dependent kinases (CDKs) bind cyclin proteins to phosphorylate and regulate retinoblastoma ( RB or MAT3 in the Volvocales), which in turn de-represses the cell cycle ( Fig. 3a ). Although most of these regulators are nearly identical in Chlamydomonas , Gonium and Volvox ( Fig. 3b,e ), there are two notable differences. First, Volvox has a four gene expansion of cyclin D1 genes ( Fig. 3c ) [17] . As Volvox has tissue differentiation, these cyclin D1 genes may have been important for tissue development as is the case in metazoans and land plants [22] , [23] , supported by the fact that RB has moved into the mating locus of Gonium and Volvox and is differentially expressed between mating loci ( Fig. 3d ) [24] , [25] . However, the tandem array expansion of the cyclin D1 genes is also found in Gonium ( Fig. 3c ), where cyclin D genes display elevated dN/dS ratios compared with other cell cycle regulators ( Supplementary Fig. 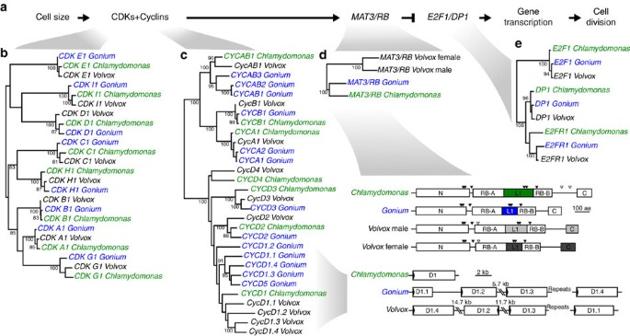8 ), suggesting the function of these cyclin Ds may be important for the transition to undifferentiated colonies, rather than tissue differentiation. Figure 3: Cell cycle pathway evolution. (a) The retinoblastoma cell cycle regulatory pathway. (b) Phylogeny of CDK genes. (c) Phylogeny of cyclin genes and syntenic relationships of cyclin D1 genes. (d) Phylogeny ofMAT3/RBgenes and comparison ofMAT3/RBproteins. Domains RB-A and RB-B, the linker region in the binding pocket (L1), N-terminal conservation (N) and C-terminal conservation (C) are shown. Difference in shade of grey forVolvoxmale andVolvoxfemale indicates sex-specific divergence24. Conserved putative CDK phosphorylation sites are indicated with solid arrows, species-specific sites are indicated with open arrows. (e) E2F/DP1 genes. All trees have a midpoint root and bootstrap values above 80% are indicated. Figure 3: Cell cycle pathway evolution. ( a ) The retinoblastoma cell cycle regulatory pathway. ( b ) Phylogeny of CDK genes. ( c ) Phylogeny of cyclin genes and syntenic relationships of cyclin D1 genes. ( d ) Phylogeny of MAT3/RB genes and comparison of MAT3/RB proteins. Domains RB-A and RB-B, the linker region in the binding pocket (L1), N-terminal conservation (N) and C-terminal conservation (C) are shown. Difference in shade of grey for Volvox male and Volvox female indicates sex-specific divergence [24] . Conserved putative CDK phosphorylation sites are indicated with solid arrows, species-specific sites are indicated with open arrows. ( e ) E2F/DP1 genes. All trees have a midpoint root and bootstrap values above 80% are indicated. Full size image Second, there is modification of the RB gene in Gonium and Volvox ( Fig. 3d , Supplementary Figs 5–7 ). Protein dimers of cyclins and CDKs primarily regulate RB by phosphorylating serine or threonine residues, which is thought to regulate RB binding of chromatin via E2F/DP transcription factors [11] , [26] , [27] . Recently it has been shown in human cells that cyclin D and CDK4/6 regulate monophosphorylation of RB proteins for G 1 phase-specific RB functions [27] . If similar in Gonium , this would suggest a role of the expanded cyclin D1 genes for regulating RB to express multicellularity-related genes during G 1 phase. If the expanded cyclin D1 proteins found in Gonium regulate multicellular cell cycle changes, modification of cyclin D-CDK phosphorylation sites in RB is predicted. Indeed, the linker of the E2F/DP binding pocket of RB is shorter in Gonium and Volvox compared with Chlamydomonas ( Fig. 3d , Supplementary Figs 5 and 6 ), potentially altering how RB binds to chromatin via E2F/DP. In addition, phosphorylation sites between the E2F/DP pocket region (RB-A and RB-B domains) and the conserved carboxy (C)-terminal domain are absent in Gonium and Volvox RB proteins ( Fig. 3d ). Interestingly, in animals the C terminus of RB is intertwined with E2F/DP and changes in the phosphorylation by cyclin–CDK complexes could also alter E2F/DP binding [28] . As these phosphorylation sites are absent in Gonium and Volvox RB proteins ( Fig. 3d ), this suggests that RB co-option for multicellularity may result in differences in locus-specific temporal expression of genes important for multicellularity during G 1 , such as cell–cell adhesion genes. Given the role the RB pathway plays in regulating the cell cycle in Chlamydomonas , its early modification found in Gonium , and its co-option for complex morphology in Volvox , RB pathway regulation might be a key step towards multicellularity in the volvocine algae. To test whether RB modifications present in Gonium and Volvox (compared with Chlamydomonas ) are unrelated to, cause or are a consequence of multicellularity, we expressed the Chlamydomonas [11] and Gonium RB genes in a Chlamydomonas strain lacking its RB gene ( rb , mat3–4 strain, Fig. 4a ) [9] , [11] using the promoter and terminator from the Chlamydomonas RB gene to ensure expression near wild-type levels ( Fig. 4b,c ) [11] . The Chlamydomonas RB gene rescues the small cell size defect in the rb mutant ( HA-CrRB::rb , Fig. 4a ), while the Gonium RB gene rescues the cell size defect and causes the Chlamydomonas rb mutant to become non-palmelloid colonial, ranging from 2 to 16 normal-sized cells ( HA-GpRB::rb , Fig. 4a ). Crossing RB gain-of-function transformed Chlamydomonas strain to a Chlamydomonas strain lacking DP1 , a gene that dimerizes with E2F to anchor RB to chromatin [11] , results in suppression of the colonial phenotype and large-sized cells ( HA-GpRB::rb::dp1 , Fig. 4a ) consistent with the phenotype of the Chlamydomonas dp1 mutant itself [10] . This demonstrates that the Gonium RB gene causes colonial multicellularity ( Fig. 4a ) through the RB pathway ( Fig. 3a ) and suggests differences in how RB binds chromatin and regulates the expression of cell cycle related genes in Gonium and Volvox are important for co-option of these RB targeted genes for multicellularity ( Figs 3 and 4 ). This gain-of-function demonstrates a causal link between cell cycle regulation and the group level during the evolution of multicellularity, emphasizing that multicellularity can evolve by co-option and modification of regulatory genes rather than extensive genomic differences or innovation. Figure 4: Gonium RB causes a colonial phenotype when expressed in Chlamydomonas . ( a ) Transformation schematic showing resulting morphology overlaid onto cell and colony size measurements (logarithmic scale) of control Chlamydomonas RB mutant ( rb or mat3 – 4 , transformed with empty vector), complementing HA-CrRB::rb (two of five independent transformations are shown) and colonial HA-GpRB::rb (four independent transformations are shown). Crossing colonial HA-GpRB::rb to a Chlamydomonas DP1 mutant ( dp1 ) restores unicellularity in Chlamydomonas (one of two independent matings are shown). ( b ) Schematic Gonium RB tagged with 3XHA with its expression driven by the Chlamydomonas RB promoter and terminator [11] . ( c ) Anti-HA immunoblotting of HA-CrRB::rb and HA-GpRB::rb with anti-tubulin loading controls. Arrows indicate proteins at their expected molecular mass. Full size image Volvox innovations for morphological complexity In Volvox , somatic differentiation is causally regulated by the regA gene cluster, a set of putative DNA-binding transcription factors thought to regulate chloroplast biogenesis [29] , [30] , [31] . The regA gene cluster is absent in Chlamydomonas and Gonium ( Fig. 5a,b ), but is present in diverse Volvox ferrisii and Volvox gigas [32] , suggesting early evolution and co-option of this cluster shortly after the split of Gonium and Volvox lineages ( Fig. 1 ) [32] . Interestingly, if the absence of regA in Gonium is indicative of the absence of regA in Astrephomene , with an independent evolution of somatic cells ( Fig. 1 ) [16] , Astrephomene may determine somatic cell fate through a different pathway than Volvox suggesting multiple evolutionary pathways and subsequent evolutionary consequences during the evolution of multicellularity. Indeed, undifferentiated multicellularity evolved once in the Volvocales [16] , while additional morphological complexity (for example, cellular differentiation and large Volvox body size) has repeatedly evolved, suggesting a relative ease to gain and lose additional complexity. 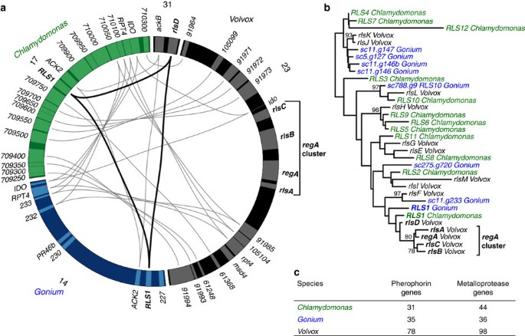Figure 5: Genetic changes present in theVolvoxgenome. (a) Gene synteny near theregAgene cluster and closely relatedregA-like genes (bold). Chromosome or scaffold number is indicated. Conserved genes are linked by line segments forregA-like (thick, black) and neighbouring genes (thin, grey). (b) Phylogenetic relationships ofregA-like genes. The tree is a midpoint root and bootstrap values above 70% are indicated. (c) Comparison of number of pherophorin and metalloprotease genes inChlamydomonas,GoniumandVolvox. Figure 5: Genetic changes present in the Volvox genome. ( a ) Gene synteny near the regA gene cluster and closely related regA -like genes (bold). Chromosome or scaffold number is indicated. Conserved genes are linked by line segments for regA -like (thick, black) and neighbouring genes (thin, grey). ( b ) Phylogenetic relationships of regA -like genes. The tree is a midpoint root and bootstrap values above 70% are indicated. ( c ) Comparison of number of pherophorin and metalloprotease genes in Chlamydomonas , Gonium and Volvox . Full size image We investigated proteins related to morphological complexity, pherophorins and matrix metalloprotease (MMP) proteins, in the volvocine algae [17] . These proteins are hypothesized to produce ECM and break up cell wall components during reproduction in Gonium and other Volvocales [15] , [33] , [34] . While Chlamydomonas contains no ECM and Gonium contains little ECM, a Volvox spheroid is largely composed of ECM ( Fig. 1 ). Pherophorin and MMP gene families are expanded in Volvox relative to Chlamydomonas ( Fig. 5c ) [17] . We found the expansion of pherophorins and MMP genes in Volvox ( Fig. 5c , Supplementary Data 2 and 3 ) is not present in Gonium , though some species-specific expansion of MMP genes has occurred ( Supplementary Data 2 and 3 ). While some expansion of ECM gene families in Gonium was expected [14] to direct the cell wall layer synthesis of a Gonium colony, this layer may instead be directed through differential gene expression. Pherophorin, MMP expansion and cellular differentiation correlate with expanded organismal size rather than the origin of multicellularity, suggesting a subsequent step in the evolution of multicellularity. We have investigated the evolution of multicellularity in the volvocine algae by sequencing the genome of the undifferentiated Gonium. Despite morphological differences, it was known that the Chlamydomonas and Volvox genomes are strikingly similar, suggesting that multicellularity required few genetic innovations [17] , [35] . However, these two genomes, positioned at the extremes of volvocine morphology, were unable to resolve the tempo and mode [36] of the evolutionary transition to multicellularity. The evolution of multicellularity in the volvocine algae is thought to involve 12 morphological innovations ( Supplementary Fig. 1 ) [15] . Five of these steps correlate with the evolution of cell groups [7] , a period of rapid evolutionary change (tempo). This view emphasizes the importance, and subsequent modification, of innovations correlating with undifferentiated colonies (mode). Finding support for this view, we have generalized these 12 steps into three major phases ( Fig. 6 ): the evolution of cell cycle regulation to form cooperative groups via cell–cell adhesion, the evolution of increased organismal size, and the evolution of differentiated germ and soma cells. Having sequenced the genome of Gonium , along with the published genomes of Chlamydomonas and Volvox , we can now identify the genetic pathways associated with each of these steps. The evolution of undifferentiated colonies correlates with RB cell cycle regulatory pathway evolution ( Figs 3 and 4 ), which is further modified as complexity increases in the Volvocales [24] . Increased organismal size toward Volvox correlates with an expansion of pherophorins and MMPs ( Fig. 5c ). Finally the evolution of the regA gene cluster underlies somatic differentiation ( Fig. 5a,b ). Future sequencing of additional Volvocales genomes should clarify the evolutionary steps required for the evolution of germ and soma. Our three-phase model for the emergence of multicellularity, supported by the genetic pathways important for their evolution, changes our understanding of the tempo and mode of multicellular evolution previously obscured in other taxa such as plants, fungi and animals due to genomic divergence ( Fig. 6 ). 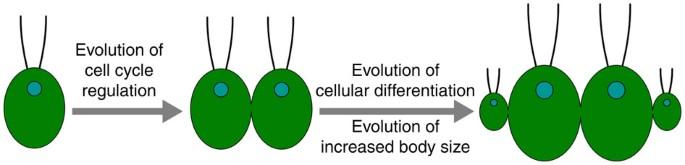Figure 6: Conceptual model for the evolution of multicellularity. Multicellularity hinges on the evolution of cell cycle regulation in a multicellular context with subsequent evolution of cellular differentiation (here, cell size-based) and increased body size. Figure 6: Conceptual model for the evolution of multicellularity. Multicellularity hinges on the evolution of cell cycle regulation in a multicellular context with subsequent evolution of cellular differentiation (here, cell size-based) and increased body size. Full size image Interestingly, an emerging theme throughout the evolution of multicellularity is that the genetic basis for the evolutionary transition emerges much earlier than anticipated [3] , [6] , [32] . In plants and animals, RB proteins are important for regulating both cell proliferation and differentiation by highly complex locus interactions with chromatin and chromatin remodelling factors [37] , [38] . Our finding that the RB pathway was co-opted early for multicellularity in undifferentiated colonies suggests that the template for subsequent evolutionary innovations in developmental programs was laid out during the transition to undifferentiated multicellularity via RB and cell cycle modifications, rather than with emergence of germ and somatic cellular differentiation. Interestingly, RB has been further co-opted for a role in sexual differentiation in Volvox , where there are male- and female-specific isoforms of RB [24] . This suggests that the evolution of multicellular cell cycle regulation was a critical step for the evolution of multicellularity. By comparing the genomes of these three volvocine green algae, we have determined that the mechanism of multicellular evolution is primarily co-option and regulatory modification of existing genetic pathways [39] . Gene duplication forms the basis of subsequent multicellular innovations. The genomic age is illuminating the genetic pathways that are important for the evolution of multicellularity in other organisms where genes such as cadherins and integrins in animals [3] , [4] and cell wall biogenesis genes in plants [6] . These are roughly analogous to metalloproteases and pherophorins in the volvocine algae highlighting convergences on similar genetic innovations for multicellularity. The substantial innovation and expansion of transcription factors and signalling networks found in animals and plants [3] , [6] is not present in the volvocine algae. However, the volvocine algae demonstrate the critical role of transcriptional regulation of the cell cycle by RB for the formation of undifferentiated colonies. RB proteins regulate the cell cycle of most eukaryotes [11] , [26] , and are tumour suppressors in humans [26] , suggesting a broader role for RB and cell cycle regulation during the evolution of multicellularity. The implications of these findings are greater than simply identifying when genes evolved during the evolution of multicellularity. Theoretical work has emphasized the need for greater understanding of the origin of an integrated group life cycle during the evolution of multicellularity [12] , [40] , [41] , [42] . The field has been concerned with the evolution of germ–soma division of labour as the defining step in the evolution of multicellularity [40] , [43] , [44] , [45] ; indeed, a recent review of animal multicellularity [45] does not mention the importance of cell cycle regulation and group formation. The Gonium genome reflects the early evolution of cell cycle regulation ( Figs 3 and 4 ) in undifferentiated groups, conserved and modified in differentiated Volvox , that is indicative of the emergence of colony level adaptations. We highlight an early and formative step, the co-option and expansion of cell cycle regulation, as important for the evolution of cooperative groups and impacting the evolution of more complicated body plans; one that may shed light on the evolutionary history of other multicellular innovations and evolutionary transitions. Strain and genome sequencing The Gonium pectorale strain K3-F3-4 (mating type minus, NIES-2863 from the Microbial Culture Collection at National Institute for Environmental Studies, Tsukuba, Japan, http://mcc.nies.go.jp/ ) was used for genome sequencing. Gonium was grown in 200–300 ml VTAC media at 20 °C with a 14:10 h light–dark cycle using cool-white fluorescent lights (165–175 μmol m −2 s −1 ). For next-generation sequencing and construction of a fosmid library, total DNA was extracted. Sequencing libraries were prepared using the GS FLX Titanium Rapid Library Preparation Kit (F. Hoffmann-La Roche, Basel, Switzerland) and the TruSeq DNA Sample Prep Kit (Illumina Inc., San Diego, CA, USA) and were run on both GS FLX (F. Hoffmann-La Roche) and MiSeq (Illumina Inc.) machines. Newbler v2.6 was used to assemble the GS FLX reads. A fosmid library was constructed in-house using vector pKS300. The fosmid library (23,424 clones) and BAC library (18,048 clones, Genome Institute (CUGI), Clemson University, Clemson, SC, USA) were end-sequenced using a BigDye terminator kit v3 (Life Technologies, Carlsbad, CA, USA) analysed on automated ABI3730 capillary sequencers (Life Technologies). Evidence-based gene prediction Introns hint file generation was done through a two-step, iterative mapping approach using Bowtie/Tophat command lines and custom Perl scripts written by Mario Stanke as part of AUGUSTUS [46] , (available at: http://bioinf.uni-greifswald.de/bioinf/wiki/pmwiki.php?n=IncorporatingRNAseq.Tophat ). AUGUSTUS version 2.6.1 was selected because its algorithm has been successfully tuned to predict genes in Chlamydomonas and Volvox genomes, which contain high GC content [46] . Reads were first mapped to the genome assembly with Tophat version 2.0.2 (ref. 47 ) and the raw alignments were filtered to create an initial (intron) hints file, which was subsequently provided to AUGUSTUS during gene prediction. An exon–exon junction database was generated from the initial AUGUSTUS prediction via a Perl script. The twice-mapped reads (once to the genome and once to the exon–exon sequences) were then merged, filtered and a final intron hints file was created. From this, the final gene prediction with AUGUSTUS was performed. Pfam domain analysis Diversity and abundance of Pfam domains was determined for all published green algae genomes. Chlorophyte genomes including Bathycoccus prasinos [48] , Chlamydomonas reinhardtii [35] , Chlorella variabilis [49] , Coccomyxa subellipsoidea C-169 (ref. 50 ), Micromonas pusilla CCMP1545 (ref. 51 ), Micromonas pusilla RCC299 (ref. 51 ), Ostreococcus tauri [52] , Ostreococcus lucimarinus [53] , Ostreococcus sp. RCC809 (US Department of Energy, Phytozome) and Volvox carteri (both versions 1 and 2; ref. 17 ) were searched using direct submission of Pfam A and Pfam B domains using Bioperl. Subsequent hits were counted and produced a matrix of Pfam domain diversity and abundance across green algae. Analysis of transcription-associated proteins Transcription-associated proteins (TAPs) include transcription factors (enhance or repress transcription) and transcription regulators (proteins which indirectly regulate transcription such as scaffold proteins, histone modification or DNA methylation). We combined three TAP classification rules for plants; PlantTFDB [54] , PlnTFDB [55] and PlanTAPDB [56] to make a set of classification rules for 96 TAP families. Conflicts between the three sets of rules were manually resolved using the rule that included more genes as transcription-associated proteins. Each transcription family includes at least one, up to three, mandatory domains. Families may include up to six forbidden domains (that is, a gene G cannot be in family F if domain D is present); not all families have defined forbidden domains. All mandatory and forbidden domains were represented by a full-length, global, Hidden Markov Model (HMM). Available HMMs were retrieved from Pfam_ls database [57] , [58] . When HMMs were not available from the Pfam_ls database, custom HMMs were made using multiple sequence alignments from PlnTFDB [55] and the HMM was calculated using HMMER version 3.0 (ref. 59 ) using ‘hmmbuild’ with default parameters and ‘hmmcalibrate—seed 0′. Gathering cutoff thresholds (GA) for the custom HMMs were set as the lowest score of a true positive hit using a ‘hmmscan’ search against several complete Chlorophyte genomes. Chlorophyte genomes including Bathycoccus prasinos [48] , Chlamydomonas reinhardtii [35] , Chlorella variabilis [49] , Coccomyxa subellipsoidea C-169 (ref. 50 ), Micromonas pusilla CCMP1545 (ref. 51 ), Micromonas pusilla RCC299 (ref. 51 ), Ostreococcus tauri [52] , Ostreococcus lucimarinus [53] , Ostreococcus sp. RCC809 (available on the DOE Phytozome website, version 10.1) and Volvox carteri [17] were searched using ‘hmmscan’ to search the library of 103 domains against the predicted protein sequences. Analyses were replicated with both Volvox version 1 and version 2; however, as results were not qualitatively different, results from version 1 are provided ( Supplementary Fig. 3 ). Subsequent hits were classified into a TAP family. Conflicts between multiple TAP families were resolved by assigning the gene to the TAP family with the highest score ( Supplementary Table 1 ). Construction of protein families Protein families were created using OrthoMCL [60] with a variety of inflation values ranging from 1.2 to 4.0 in steps of 0.1 ( Supplementary Figs 16–17 ). This analysis was performed using Chlorophyte genomes available on the DOE JGI Phytozome website, version 10.1 including Bathycoccus prasinos [48] , Chlamydomonas reinhardtii [35] , Chlorella variabilis [49] , Coccomyxa subellipsoidea C-169 (ref. 50 ), Micromonas pusilla CCMP1545 (ref. 51 ), Micromonas pusilla RCC299 (ref. 51 ), Ostreococcus tauri [52] , Ostreococcus lucimarinus [53] , Ostreococcus sp. RCC809 (available on the DOE Joint Genome Institute website) and Volvox carteri [17] . This analysis was repeated for both Volvox version 1 and Volvox version 2. The inflation value of 1.9 was used for both analyses for consistency and was chosen to have relatively large, coarser grained clusters that were robust to higher inflation values ( Supplementary Figs 16–19 ). To avoid bias introduced by not including all genes for each species, genes not assigned to a gene family (singletons) were assigned to single gene families and included in all subsequent phylogenetic gene family analyses. A species tree was calculated by extracting OrthoMCL gene families containing only one copy in each species, for a total of 1,457 genes. The OrthoMCL run with an inflation value of 1.5 was chosen to use larger, coarser grained clusters, thus increasing the likelihood of capturing true 1:1:1 orthologues. This species tree included Volvox carteri version 2. These genes were independently aligned using Muscle version 3.8.31 (ref. 61 ) and concatenated. A phylogenetic tree was produced using RAxML version 8.0.20 (ref. 62 ) using the Protein Gamma model with automatic model selection on a per gene basis via partitions for each protein. A rapid bootstrapping analysis to search for the best-scoring ML tree was run with 100 bootstraps. The resulting species tree is consistent with previous results [16] , [51] , [63] , [64] , [65] and had 100 bootstrap support at every node ( Supplementary Fig. 20 ). This result is also consistent with numerous morphological characteristics supporting a closer relationship of Gonium and Volvox [66] . Gene family evolution within the volvocine algae was analysed using Count version 10.04 (ref. 67 ) to perform several parsimony analyses including symmetric Wagner parsimony (each gene family may be gained or expanded multiple times and the gain penalty is equal to the loss penalty) and asymmetric Wagner parsimony (each gene family may be gained or expanded multiple times and the gain penalty is two times higher than the loss penalty). This analysis was repeated for both Volvox version 1 and version 2 genomes ( Supplementary Tables 5–8 ). dN/dS analysis During our OrthoMCL construction of protein gene families, we identified 6,154 clusters with exactly one copy in Chlamydomonas (version 5.3), Gonium and Volvox (version 2). The number of genes from other unicellular (non- Chlamydomonas ) Chlorophyte species was ignored. This criteria is relatively strict as it does not include any genes with a duplicate in any species (copy number greater than one in any species) or any genes which are not essential (no copy present in any species) resulting in 1:1:1 orthologues. Given the relatively high gene duplication rates in volvocine algae (data not shown), these strict criteria support an interpretation of 1:1:1 orthology. Genome-wide pairwise comparisons of dN, dS and dN/dS were calculated ( Supplementary Fig. 21 ; Supplementary Table 11 ) using PAML and codeml (ML analysis [68] ) based on nucleotide translation based alignments (proteins were aligned using MUSCLE [61] ). Prediction of lineage-specific genes The phylostratigraphy method [20] assumes Dollo’s parsimony (that is, it is more likely that a gene observed in two distant clades was present in the common ancestor and multiple independent gains are not possible). This provides an entry point for testing evolutionary hypotheses related to the age of genes and to quantify how much gene-level innovation has occurred along each phylogenetic branch. Old genes are classified in low phylostrata (present in distant species, PS1–PS7) and young genes are classified in higher phylostrata (for example, genus- or species-specific genes, PS8–PS9). The resolution of each phylostratum strictly depends on the availability of reliable outgroups (the availability of reliable genomic outgroups is relatively low in Chlorophyte algae). The phylogenetic classes were defined from those in each NCBI Taxonomy entry for Chlamydomonas , Gonium and Volvox , resulting in nine expected phylostrata for each species. All proteins were subjected to a BLASTP search with an E -value threshold of 0.001 against the NCBI nr database. Placement in phylostrata was derived from the taxonomic information of these hits for each protein, using the most distant hit, and following Dollo’s parsimony. Phylogenetic analyses Unless otherwise stated, all phylogenetic analyses were performed using a custom pipeline of SATe version 2.2.7 (ref. 69 ) coupled with RAxML version 8 (ref. 62 ). Full gene protein sequences were passed to SATe using a FASTTREE tree estimation with a RAxML search after tree formation with a maximum limit of 10 iterations and the ‘longest’ decomposition strategy. Bootstraps were made on the SATe output alignment and tree using RAxML with automatic model selection, a rapid hill climbing algorithm (−f d) and 100 bootstrap partitions. Bipartition information (−f a) was obtained using the SATe output tree and RAxML bootstraps. Chlamydomonas strains culture conditions Wild-type Chlamydomonas reinhardtii 6145 and 21gr, and HA-CrRB ( HA-MAT3::mat3–4 , here referred to as HA-CrRB::rb ), mat3–4 (here referred to as rb ), and dp1 have been previously described [9] , [10] , [11] . Briefly, wild-type strains 6145 (MT−) and 21gr (MT+) are mating pairs that have been back crossed to eliminate the y1 mutation in 6145 (ref. 10 ). The RB knockout strain has been previously characterized as a null allele, and the knockout mutation is the rb allele [9] , [11] . The rb mutation can be complemented by a amino (N)-terminally tagged version of the gene that behaves identical to wild type. Previously, a knockout mutation in the Chlamydomonas DP1 gene, dp1 , was identified and characterized [10] , [11] . All the strains were maintained on TAP plates. For phenotype analysis, the strains were grown in high salt media (HSM) synchronously under 14 h of 150 μE of light, samples were fixed hourly and examined by light microscopy [10] , [11] . Cloning of Gonium pectorale RB and transformation into rb A 3X haemagluttin (HA) tagged copy of the Gonium pectorale RB gene was cloned using InFusion Cloning (Clontech) to be driven by the Chlamydomonas RB promoter and terminator that includes a AphVIII selectable marker for Chlamydomonas transformation ( Fig. 4 , (ref. 11 )). Gonium pectorale genomic DNA from K4F3 was used as a template and the genomic region of RB was amplified without its ATG start codon using the primers 5′-CAGATTACGCTACTAGATCTGCCGAAGCTGAACGTTTTACTGCG-3′, and 5′-CTCCGGCCGCGGTGCCTAATTTGCGCCGTACCGCCGGA-3′. These primers overlap with the 3X HA tag and 3′ terminator from the previously created HA-CrRB transformation clone that complements the rb mutation [11] . The HA-CrRB plasmid was amplified by inverse PCR with 5′-TCTAGTAGCGTAATCTGGAACGTCATATGGATAGG-3′ and 5′-GCACCGCGGCCGGAGGT-3′ primers. PCR products were gel purified with a QiaQuick gel extraction kit (Qiagen). Purified PCR fragments were fused by InFusion (Clontech) cloning based on overlaps in the amplified sequences and transformed into chemically competent DH5-apha cells, after which the clone was confirmed by sequencing. Transformation of Chlamydomonas reinhardtii The rb strain was transformed with glass beads [11] , with the HA-GpRB clone (above) and as a control with HA-CrRB and pSI103 ( AphVIII selectable marker only) and selected on TAP plates supplemented with 20 μg ml −1 paromycin [11] . Candidate strains were screened by growth morphology [10] , [11] , and then screened for expression by immunoblotting with an anti-HA antibody (Roche 3F10, high affinity [11] ). Four independent strains expressing the HA-GpRB , and five independent strains expressing HA-CrRB were created. Control complementation of the rb mutation with HA-CrRB occurred at rates similar to previous results [11] . The presence of the rb mutation was confirmed by replica plating on TAP plates supplemented with 10 μg ml −1 emetine [9] , [11] . Genetic analysis of HA-GpRB -expressing strains Two lines expressing HA-GpRB were crossed to a dp1 null mutation [10] . Because both the HA-GpRB and dp1 mutations are linked to AphVIII, single tetrads were dissected. HA-GpRB was genotyped with primers in the 3XHA tag 5′-AGTGCTAACAGCATGTCTAGTTAC-3′, and in the 5′ portion of GpRB 5′-TGCGAACAACCGCTGCAGACCTTC-3′. The dp1 mutation was genotyped as previously described [10] . Immunoblotting HA-GpRB and HA-CrRB strains complementing rb Whole-cell lysates from strains were prepared, separated and immunoblotted [11] . Briefly, the anti-HA antibody used for detection of HA-GpRB and HA-CrRB was an anti-HA high affinity monoclonal antibody (clone 3F10, Roche) and anti-alpha-tubulin monoclonal antibody (Sigma), as previously described [11] . The expression levels of RB in HA-CrRB strains have been previously shown to be similar to wild-type Chlamydomonas expression levels [11] . The expression levels of RB in HA-GpRB are similar, if not slightly below, the expression levels of HA-CrRB , suggesting that overexpression of RB is not causing the observed colonial phenotype, but rather modification to the Gonium RB gene. Measurement of cell or colony size distribution The size of cells and groups of cells was measured with a Moxi Z automated cell sizer/counter using type ‘S’ cassettes (ORFLO Technologies). Sizing is based on the Coulter principle used previously with Chlamydomonas reinhardtii [10] , [11] . Accession codes: This Whole Genome Shotgun project has been deposited at DDBJ/ENA/GenBank under the accession LSYV00000000 . The version described in this paper is version LSYV01000000 . Data are also available via JGI Phytozome. How to cite this article: Hanschen, E. R. et al. The Gonium pectorale genome demonstrates co-option of cell cycle regulation during the evolution of multicellularity. Nat. Commun. 7:11370 doi: 10.1038/ncomms11370 (2016).